Quantum-coupled radial-breathing oscillations in double-walled carbon nanotubes Van der Waals-coupled materials, ranging from multilayers of graphene and MoS 2 to superlattices of nanoparticles, exhibit rich emerging behaviour owing to quantum coupling between individual nanoscale constituents. Double-walled carbon nanotubes provide a model system for studying such quantum coupling mediated by van der Waals interactions, because each constituent single-walled nanotube can have distinctly different physical structures and electronic properties. Here we systematically investigate quantum-coupled radial-breathing mode oscillations in chirality-defined double-walled nanotubes by combining simultaneous structural, electronic and vibrational characterizations on the same individual nanotubes. We show that these radial-breathing oscillations are collective modes characterized by concerted inner- and outer-wall motions, and determine quantitatively the tube-dependent van der Waals potential governing their vibration frequencies. We also observe strong quantum interference between Raman scattering from the inner- and outer-wall excitation pathways, the relative phase of which reveals chirality-dependent excited-state potential energy surface displacement in different nanotubes. Electronic and vibrational coupling in the nanoscale governs many important physical processes, such as energy transfer in photosynthesis [1] , charge separation in heterojunctions [2] and thermal transport through interfaces [3] . Quantum coupling between nanostructures is also crucial for understanding emerging properties in van der Waals-coupled superstructures, such as multilayer of graphene and superlattice of nanoparticles. Double-walled carbon nanotubes (DWNTs), a coaxial composite of two single-walled carbon nanotubes (SWNTs), provide a unique model system for quantitative study of such nanoscale coupling, because the structural and physical properties of DWNTs are precisely defined individually, but richly varied among different species [4] , [5] , [6] , [7] , [8] , [9] , [10] , [11] , [12] . Specifically, a SWNT is uniquely defined by its chiral indices ( n , m ). A DWNT, composed of two SWNTs, is fully defined by chiral indices ( n o , m o )/( n i , m i ) of the coaxial outer-/inner-walls [10] , [11] , [12] . Its electronic and vibrational properties, however, can differ profoundly from those of the constituent SWNTs owing to tube–tube interactions. Radial-breathing mode (RBM) oscillation is a signature vibration of one-dimensional nanostructures. It is widely used for characterizing carbon nanotubes [13] , [14] , [15] , [16] , [17] , and can be sensitively measured at the single-nanotube level using resonance Raman spectroscopy [18] , [19] , [20] . In SWNTs, the RBM oscillation frequency ( ω RBM ) uniquely determines the nanotube diameter ( D ) following a simple scaling law ω RBM =228/ D (nm cm −1 ) [21] . The RBM behaviour in DWNTs, however, is drastically different owing to strong inter-tube coupling. The coupling effects in DWNTs have been actively investigated for over one decade [4] , [5] , [6] , [7] , [8] , [9] , but they are still poorly understood. In this letter, we systematically study quantum-coupled RBM oscillations in chirality-defined DWNTs by simultaneously determining structural, electronic and vibrational properties of individual nanotubes with combined single-tube electron diffraction [11] , [12] , Rayleigh scattering [22] , [23] and Raman scattering [18] , [19] , [20] techniques. We show that mechanical coupling between the walls lead to collective oscillation modes with concerted inner- and outer-wall vibrations in DWNTs. Oscillation frequencies of the coupled RBM modes can be quantitatively described by a coupled oscillator model, where the coupling originates from the van der Waals force between the inner and outer tubes. Different DWNTs, which have different inner- and outer-wall separations, allow us to probe the inter-tube van der Waals interactions at an effective pressure that can be both positive and negative and at gigapascal level. The coupled RBM oscillations also exhibit unusual electron–phonon interactions. They always appear in pairs in resonance Raman spectra, because each RBM mode couples to electronic resonances in both walls. Furthermore, Raman amplitudes from inner- and outer-wall excitation channels can interfere quantum mechanically. Relative interference phase between the two Raman channels enabled us to examine the displaced excited-state potential energy surface in SWNTs and its dependence on the nanotube chirality. 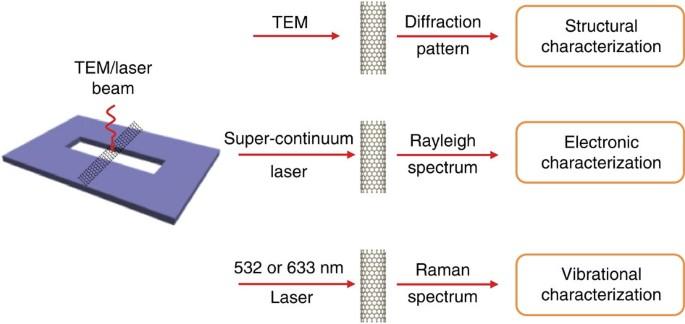Figure 1: Schematic illustration of the experimental design. The substrate is etched with open slit, where individual suspended nanotubes are directly grown on. TEM beam and laser beam can both go through the slit. This design enables the combination of TEM electron diffraction, Rayleigh scattering and Raman scattering techniques to, respectively, probe the structural, electronic and vibrational properties of the same individual carbon nanotubes. Experimental design Figure 1 shows the schematic illustration of our experimental design. We utilized the SiO 2 /Si wafer with open slit as our base substrate, where suspended carbon nanotubes are directly grown on (See Methods for more details). Transmission electron microscope (TEM) beam and laser beam can both go through the slit. This design enables the combination of TEM electron diffraction, Rayleigh scattering and Raman scattering techniques to probe the structural, electronic and vibrational properties of the same individual nanotubes. In addition, the use of the as-grown suspended nanotubes makes to exclude the substrate effects and ensures to probe the intrinsic physical properties of carbon nanotubes. Figure 1: Schematic illustration of the experimental design. The substrate is etched with open slit, where individual suspended nanotubes are directly grown on. TEM beam and laser beam can both go through the slit. This design enables the combination of TEM electron diffraction, Rayleigh scattering and Raman scattering techniques to, respectively, probe the structural, electronic and vibrational properties of the same individual carbon nanotubes. 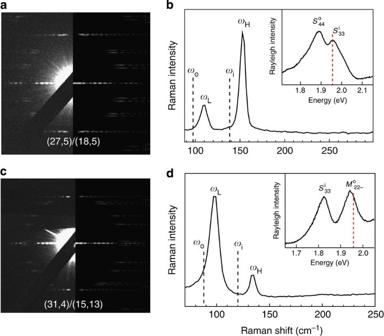Figure 2: Coupled radial-breathing mode vibrations in double-walled carbon nanotubes. (a,b) TEM electron diffraction pattern and Raman spectrum for DWNT (27, 5)/(18, 5). Two well-defined RBM peaks are present in the Raman spectrum, and their frequencies are strongly blue-shifted from those of the constituent single-walled nanotubes (indicated by dashed lines). The excitation photon energy of 1.96 eV is in resonance with both inner-walland outer-wallelectronic transitions, as shown in the Rayleigh scattering spectrum (inset ofb). (c,d) TEM electron diffraction, Raman and Rayleigh spectrum data for the (31, 4)/(15, 13) DWNT. Two appreciably blue-shifted RBM oscillations are again observed. In this DWNT, Raman excitation energy (1.96 eV) is only in resonance with thetransition of the metallic outer-wall nanotube. Full size image Coupled RBM vibrations in DWNTs Figure 2 displays electron diffraction patterns, Rayleigh scattering and Raman scattering spectra for two representative individual DWNTs. Electron diffraction patterns ( Fig. 2a ) unambiguously determine the DWNT chiral indices ( n o , m o )/( n i , m i ) to be (27, 5)/(18, 5) and (31, 4)/(15, 13). Electronic transitions of the two DWNTs are obtained from the Rayleigh scattering spectra (insets in Fig. 2b , respectively), in which prominent optical resonances can be observed. By comparing the optical resonances in Rayleigh spectra of DWNTs to that of the constituent SWNTs, we can assign the resonance peaks to inter-subband electronic transitions of either inner- and outer-wall nanotubes because tube–tube interactions in DWNTs produces only a small shift (tens of meV) of the electronic transition energies [24] . We measure the RBM oscillations of DWNTs using resonant Raman scattering. Two well-defined RBM peaks are observed in the resonant Raman spectra of the (27, 5)/(18, 5) and (31, 4)/(15, 13) DWNTs ( Fig. 2b ). The laser excitation energy (1.96 eV) is marked by dashed line in the figure insets showing the Rayleigh scattering spectra. We have studied 35 DWNTs with well-defined Rayleigh scattering resonances (that can be assigned to each tube components) and TEM diffraction data. Of these DWNTs, 13 have one or more electronic transitions in resonance with our Raman excitation lasers. RBM Raman peaks are observed in, and only in, these 13 tubes. We summarized in Table 1 their chirality and Raman data. Our DWNTs have relatively large diameters, with inner-wall diameter ( D i ) >1.5 nm in all the nanotubes. Figure 2: Coupled radial-breathing mode vibrations in double-walled carbon nanotubes. ( a , b ) TEM electron diffraction pattern and Raman spectrum for DWNT (27, 5)/(18, 5). Two well-defined RBM peaks are present in the Raman spectrum, and their frequencies are strongly blue-shifted from those of the constituent single-walled nanotubes (indicated by dashed lines). The excitation photon energy of 1.96 eV is in resonance with both inner-wall and outer-wall electronic transitions, as shown in the Rayleigh scattering spectrum (inset of b ). ( c , d ) TEM electron diffraction, Raman and Rayleigh spectrum data for the (31, 4)/(15, 13) DWNT. Two appreciably blue-shifted RBM oscillations are again observed. In this DWNT, Raman excitation energy (1.96 eV) is only in resonance with the transition of the metallic outer-wall nanotube. Full size image Table 1 Chiral indices and coupled radial-breathing mode oscillation data for double-walled carbon nanotubes. Full size table There are two striking features in the RBM Raman data of these (relatively large diameter) DWNTs. (1) Frequencies of the two RBM oscillations in DWNTs, denoted as ω L and ω H , are respectively much higher than the RBM frequencies of the constituent outer-( ω o ) and inner-wall SWNTs ( ω i ) (for example, Fig. 2b ). If this blue shift is attributed to a simple increase of ‘effective’ restoration force, this restoration force has to increase by as high as 35%. (2) The resonant peaks almost always appear in pairs in resonant Raman spectra: there are either no RBM peak (in 21 tubes) or two RBM peaks (in 13 tubes). Only one nanotube has just one RBM peak. This behaviour is quite surprising, because conventional picture suggests that resonance enhancement of the inner- and outer-wall RBM oscillations are largely independent [5] , [7] and most nanotubes should have a single RBM peak when excited resonantly. To understand the unusual RBM behaviour in DWNTs, we have to realize that tube–tube interactions in these DWNTs are not small perturbations. Instead, they qualitatively change the DWNT RBM oscillations by strongly mixing the inner- and outer-wall vibrations: the observed lower-( ω L ) and higher-frequency ( ω H ) RBM modes are collective oscillations with concerted in-phase and out-of-phase motion of the two walls. Inter-wall van der Waals interactions in DWNTs The collective RBM oscillations of a unit-length DWNT can be modelled by a coupled mechanical oscillator with five parameters: m i , k i , m o , k o and k c ( Fig. 3a ) [25] . The unit-length mass of the inner- and outer-walls ( m i and m o ) can be obtained directly from the tube chiral indices, and the unit-length intrinsic force constant of the two walls ( k i and k o ) can be obtained from RBM frequencies of isolated SWNTs ( Supplementary Note S1 ). The only unknown parameter is the coupling force constant k c , which characterizes the van der Waals interaction between the two walls of the DWNT. Using a single value of k c for any given DWNT, we can simultaneously reproduce the in-phase ( ω L ) and out-of-phase RBM vibration frequencies ( ω H ) ( Fig. 3b ). For different DWNTs, the coupling constant k c vary significantly. 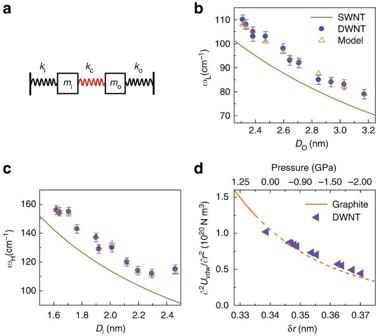Figure 3: Coupled nanomechanical oscillations in double-walled carbon nanotubes. (a) Illustration of the coupled oscillator model, wheremi(mo) andki(ko) are, respectively, the inner(outer)-wall nanotube unit-length mass and intrinsic force constant, andkcis the unit-length coupling force constant owing to tube–tube interactions. (b) Lower RBM frequencies of the DWNTs versus outer-wall nanotube diameters (dots), which are appreciably higher than uncoupled out-wall nanotube RBM frequencies (line). Theoretical prediction based on the coupled oscillator model (triangles) agrees well with our data. (c) Higher RBM frequencies of the DWNTs versus inner-wall nanotube diameters, which display analogous behaviour as in (b). The error bar in (b) and (c) represents the uncertainty in fitting the RBM resonance in Raman spectra. (d) Derived unit-area force constant owing to tube–tube van der Waals interaction, ∂2Uvdw/∂r2, for different inter-tube separation (triangles), and the comparison to results from high-pressure graphite measurements (line). The different inter-tube separation in DWNTs corresponds an effective pressure variation from 0.2 to −2.0 GPa (top label). (The zero-pressure inter-tube distance for DWNTs is slightly shifted from that of graphite owing to the finite tube curvature4). Figure 3: Coupled nanomechanical oscillations in double-walled carbon nanotubes. ( a ) Illustration of the coupled oscillator model, where m i ( m o ) and k i ( k o ) are, respectively, the inner(outer)-wall nanotube unit-length mass and intrinsic force constant, and k c is the unit-length coupling force constant owing to tube–tube interactions. ( b ) Lower RBM frequencies of the DWNTs versus outer-wall nanotube diameters (dots), which are appreciably higher than uncoupled out-wall nanotube RBM frequencies (line). Theoretical prediction based on the coupled oscillator model (triangles) agrees well with our data. ( c ) Higher RBM frequencies of the DWNTs versus inner-wall nanotube diameters, which display analogous behaviour as in ( b ). The error bar in ( b ) and ( c ) represents the uncertainty in fitting the RBM resonance in Raman spectra. ( d ) Derived unit-area force constant owing to tube–tube van der Waals interaction, ∂ 2 U vdw /∂ r 2 , for different inter-tube separation (triangles), and the comparison to results from high-pressure graphite measurements (line). The different inter-tube separation in DWNTs corresponds an effective pressure variation from 0.2 to −2.0 GPa (top label). (The zero-pressure inter-tube distance for DWNTs is slightly shifted from that of graphite owing to the finite tube curvature [4] ). Full size image The tube-dependent k c provides a unique way to examine how the van der Waals interaction varies with the separation between the inner- and outer-wall tubes. The unit-length coupling force constant kc can be expressed approximately using the average unit-area inter-tube van der Waals potential U vdw with , where the mean diametre . In our as-grown DWNTs, the separation between the inner- and outer-tubes δr =( D o − D i )/2 can vary from 0.34 to 0.37 nm, which is uniquely determined by the tube chiral indices. Figure 3d displays the data for unit-area force constant part; 2 U vdw / part;r 2 , which changes by over two times over the range of inter-tube separation existing in our DWNTs. Our results can be compared with the van der Waals interaction between unit-area graphene sheets under pressure obtained from compressibility measurements of graphite (solid line) and theoretical extrapolation in the negative pressure range (dashed line) [26] , and they agree well. This comparison shows that the effective pressure between the walls of as-grown DWNTs reaches gigapascals owing to variations in the tube–tube separation [26] , [27] . It is interesting to note that DWNTs allow us to readily access a negative pressure in the gigapascal range, which is difficult to achieve using conventional approaches. The force constant deduced here is related to the C 33 modulus of graphite, and its value is about one order of magnitude larger than that from the shear mode of few-layered graphene, which is related to the C 44 modulus of graphite [28] , [29] . Quantum interference in resonance Raman process in DWNTs Unlike separated inner- and outer-SWNTs RBM excitations (illustrated in Fig. 4a ), the collective DWNT oscillations ω L and ω H contain both inner- and outer-wall motion, and they couple simultaneously to electronic transitions in both walls ( Fig. 4b ). Therefore, both coupled RBM oscillations will be resonantly excited if an electronic transition of either wall matches the excitation photon energy. This leads to the unusual behaviour that we observed experimentally: the RBM Raman modes are mostly either not observable (in 21 tubes) or appearing in pairs (in 13 tubes) in resonant Raman scattering spectra of DWNTs. 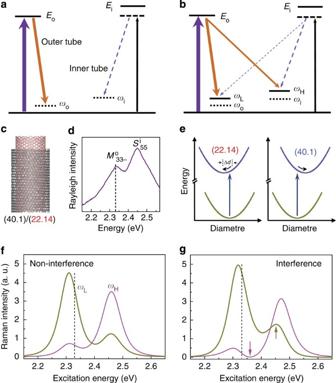Figure 4: Quantum interference in resonance Raman process in double-walled carbon nanotubes. (a) Raman process with non-coupled outer and inner SWNT oscillations. The radial breathing mode (RBM) vibration of the SWNT exhibits strong Raman scattering when electronic transition resonant with excitation photon energy. Therefore, resonance Raman peaks for outer- and inner-SWNT appear independently. (b) Raman process with collective outer- and inner-wall oscillations. The coupled oscillations have higher frequencies, and each of them couples to both inner- and outer-SWNT electronic transitions. Resonance Raman peaks always appear in pairs even when only one electronic transition is in resonance. In addition, the vibrations from the inner- and outer-wall excitation channels will interfere with each other quantum mechanically. (c) Atomic model of DWNT (40, 1)/(22, 14). (d) Rayleigh spectrum of DWNT (40, 1)/(22, 14). The 2.33 eV Raman photon excitation is resonant with the outer-wall metallictransition but not the inner-wall semiconductingtransition, therefore two walls have opposite resonance phase factors. (e) The potential energy surfaces for theandexcited states in the constituent (22, 14) and (40, 1) SWNTs. The displacements (Δd) are extremely small at ~1 fm, and they are exaggerated in the figure for illustration. The photo-induced RBM vibration can be understood in the Frank–Condon picture. Upon optical excitation the SWNT lattice, starting from the equilibrium configuration of the ground state, relaxes based on the excited-state potential energy surface and sets off the RBM vibration. (f,g) Simulated Raman intensities of out-of-phase (ωH) and in-phase (ωL) RBM modes versus excitation laser energy for the (40, 1)/(22, 14) DWNT without (f) and with (g) the quantum interference. The opposite resonance phase factors of the two walls (d), together with the oppositely displaced excited potential energy surfaces (e), will drive the inner- and outer-walls to vibrate mostly in the same direction after the optical excitation, and enhance the in-phase oscillationωLwhile suppress the out-of-phase oscillationωHowing to quantum interference (g). It leads to significantly enhanceIL/IHat our Raman excitation energy 2.33 eV (dashed line), as observed experimentally. Figure 4: Quantum interference in resonance Raman process in double-walled carbon nanotubes. ( a ) Raman process with non-coupled outer and inner SWNT oscillations. The radial breathing mode (RBM) vibration of the SWNT exhibits strong Raman scattering when electronic transition resonant with excitation photon energy. Therefore, resonance Raman peaks for outer- and inner-SWNT appear independently. ( b ) Raman process with collective outer- and inner-wall oscillations. The coupled oscillations have higher frequencies, and each of them couples to both inner- and outer-SWNT electronic transitions. Resonance Raman peaks always appear in pairs even when only one electronic transition is in resonance. In addition, the vibrations from the inner- and outer-wall excitation channels will interfere with each other quantum mechanically. ( c ) Atomic model of DWNT (40, 1)/(22, 14). ( d ) Rayleigh spectrum of DWNT (40, 1)/(22, 14). The 2.33 eV Raman photon excitation is resonant with the outer-wall metallic transition but not the inner-wall semiconducting transition, therefore two walls have opposite resonance phase factors. ( e ) The potential energy surfaces for the and excited states in the constituent (22, 14) and (40, 1) SWNTs. The displacements (Δ d ) are extremely small at ~1 fm, and they are exaggerated in the figure for illustration. The photo-induced RBM vibration can be understood in the Frank–Condon picture. Upon optical excitation the SWNT lattice, starting from the equilibrium configuration of the ground state, relaxes based on the excited-state potential energy surface and sets off the RBM vibration. ( f , g ) Simulated Raman intensities of out-of-phase ( ω H ) and in-phase ( ω L ) RBM modes versus excitation laser energy for the (40, 1)/(22, 14) DWNT without ( f ) and with ( g ) the quantum interference. The opposite resonance phase factors of the two walls ( d ), together with the oppositely displaced excited potential energy surfaces ( e ), will drive the inner- and outer-walls to vibrate mostly in the same direction after the optical excitation, and enhance the in-phase oscillation ω L while suppress the out-of-phase oscillation ω H owing to quantum interference ( g ). It leads to significantly enhance I L / I H at our Raman excitation energy 2.33 eV (dashed line), as observed experimentally. Full size image The collective RBM oscillations in DWNTs couple to the electronic excitations quantum mechanically, and it leads to interesting quantum interference between the inner- and outer-wall excitation pathways. With such quantum interference even non-resonant contribution can become important, and Raman intensities of the coupled RBM oscillations in DWTNs are described by the superposition of Raman amplitudes from inner- and outer-wall excitation pathways as Here, ‹ ω i(o) | ω L(H) › is the inner(outer)-wall component of the coupled RBM mode ω L ( ω H ), and its value can be calculated directly from a quantized coupled mechanical oscillator model illustrated in Fig. 3a ( Supplementary Note S2 ). R i(o) and M i(o) denotes, respectively, the electronic resonance factor and Raman matrix element of the inner(outer)-wall SWNT excitations. The resonance factor R i(o) can be obtained from Rayleigh scattering spectra of the DWNTs, which probe directly the optical resonances of both the inner- and outer-wall nanotubes ( Supplementary Note S3 ). The Raman matrix element M i(o) characterizes how the phonon couples to the photo-excited exciton in the inner(outer)-wall nanotube. For simplicity, we will assume that M i and M o have the same magnitude and focus on their relative sign, s =sgn( M i / M o ). This simplification emphasizes the importance of the phase factor, which determines whether the quantum interference is constructive or destructive for the coupled RBM oscillations. To compare with the experiment quantitatively, we use the Raman intensity ratio I L / I H because it does not depend on an absolute determination of Raman cross-section. The ratio has the form of in our approximation. In Table 1 , we listed the measured Raman intensity ratio ( I L / I H ) exp together with calculation results including the quantum interference ( I L / I H ) I and not including the interference ( I L / I H ) N−I . Nice agreement between the theory and experiment is achieved when, and only when, the quantum interference effect is fully included using the correct s parameter. We take a closer look at the Raman quantum interference using (40, 1)/(22, 14) DWNT as an example ( Fig. 4c ). The s parameter, which characterizes the relative sign between Raman matrix elements M i and M o , depends sensitively on the chirality of the inner- and outer-SWNTs. Its value is related to the relative motion direction of the inner- and outer-wall nanotubes immediately after the optical excitation. A physical picture of this process in outer- and inner-SWNTs is provided by recalling Frank–Condon effects ( Fig. 4e ): the excited state has a displaced potential energy surface compared with that of the ground state. The displacement is extremely small (~1 fm), but is essential for the exciton–phonon coupling. Upon optical excitation, the SWNT lattice, initially at the ground-state equilibrium configuration, relaxes based on the excited-state potential energy surface and sets off the RBM vibration. In (40, 1)/(22, 14) DWNT the potential energy surface displacements of inner- and outer-walls displace are opposite with an s =−1 (refs [30] , [31] 30,31). To determine the RBM oscillation interference, we also need to include the resonance phase factor. For (40, 1)/(22, 14) DWNT, the phase factors are nearly opposite for the (non-resonant) inner- and (resonant) out-wall pathways with 2.33 eV photon excitation ( Fig. 4d ). The opposite resonance phase factors, together with s =−1, determine that the quantum interference will suppress the Raman intensity of ω H while enhance that of ω L. This quantum interference leads to increased I L / I H ratio from 5.8 to 20, and the experimental value of I L / I H is 19 ( Table 1 ). We further plot the calculated RBM Raman intensity of the (40, 1)/(22, 14) DWNT at different excitation energies without ( Fig. 4f ) and with the quantum interference ( Fig. 4g ), which displays the variation of quantum interference effects with the excitation laser energy. Our observed s parameter shows that the relative displacement of the excited-state potential energy surface varies with the SWNT chirality, and it can be described by a simple family pattern: the excited-state potential energy surface is displaced inwards for transitions on one side of the zig–zag cut through K point of the graphene Brillouin zone, which includes even transitions of mod( n − m ,3)=1 semiconducting, odd transitions of mod( n − m ,3)=2 semiconducting and higher branch transitions of non-armchair metallic nanotubes. The displacement is outwards for all other transitions. This is the first observation of family behaviour in the excited-state potential energy surface displacement, which has been predicted previously theoretically in ab initio and tight-binding calculations [30] , [31] . The ability to combine structural, electronic and vibrational characterization on the same individual DWNTs allows us to systematically investigate quantum-coupled mechanical oscillations and their unusual interactions with electronic excitations for the first time. We show that van der Waals interaction, usually treated as a weak perturbation, can actually produce quantum phenomena in coupled nanostructures that have only been observed in covalent material previously. With exact structural determination, we are able to determine the separation-dependent van der Waals coupling between nanotube walls and the excited-state potential energy surfaces of constituent nanotubes. Such approach can also be used to explore other composite nanostructures. It will enable quantitative understanding of van der Waals interactions and the electronic and vibrational couplings in the nanoscale. In our experiment, we use suspended DWNTs that are free of substrate effects and compatible with both TEM and single-tube optical spectroscopy techniques. Long suspended nanotubes were grown by chemical vapour deposition (CVD) across open slit structures (~30 × 500 μm) fabricated on silicon substrates [32] . We use Fe nanoparticles as catalysts and methane in hydrogen (CH 4 :H 2 =1:2) as gas feedstock, and control the size of catalyst particles to achieve the selective abundance of DWNTs [33] . We determine chiral structures of DWNTs using electron diffraction with nano-focused 80 keV electron beams in a JEOL 2100 TEM [11] , [12] . Utilizing the slit edges as markers, the same individual nanotubes can be identified in an optical microscopy setup. To determine electronic transitions of these individual nanotubes, we use Rayleigh scattering spectroscopy with a fibre-laser-based supercontinuum light source covering the spectral range from 450 to 900 nm (refs [22] , [23] 22,23). To determine RBM vibration and electron–phonon coupling in these individual nanotubes, we use resonant Raman scattering spectroscopy with laser excitation at photon energy of 1.96 or 2.33 eV (refs [18] , [19] , [20] 18–20). Our instrumental resolution for RBM Raman frequency is ~2 cm −1 . How to cite this article: Liu, K. et al. Quantum-coupled radial-breathing oscillations in double-walled carbon nanotubes. Nat. Commun. 4:1375 doi: 10.1038/ncomms2367 (2012).